Doubly N-confused and ring-contracted [24]hexaphyrin Pd-complexes as stable antiaromatic N-confused expanded porphyrins As isomers of the regular porphyrins, N-confused porphyrins have attracted extensive attention of chemists because of their unique chemical structures, chemical reactivities, and physical properties, which result in their promising applications in the fields of catalytic chemistry, biochemistry and material science. Typically, N-confused porphyrins are synthesized via acid catalyzed condensation and following oxidation during which lactams are often formed as the byproducts. Here we report doubly N-confused and ring-contracted [24]hexaphyrin(1.1.0.1.1.0) mono- and bis-Pd-complexes as stable antiaromatic N-confused expanded porphyrins, which are synthesized through Pd-catalyzed Suzuki-Miyaura coupling of 1,14-dibromotripyrrin. These macrocycles show a paratropic ring currents, an ill-defined Soret band, a red-shifted weak absorption tail, and a small HOMO-LUMO gap. NBS bromination of the bis Pd-complex give its mono- and dibromides regioselectively, which are effectively used to synthesize a [24]hexaphyrin dimer and a Ni II porphyrin-[24]hexaphyrin-Ni II porphyrin triad, respectively. In the chemistry of porphyrinoids, expanded porphyrins [1] , [2] , [3] , [4] , [5] and N-confused porphyrins (NCPs) [6] , [7] , [8] , [9] are two important newcomers, which have contributed to highlighting the glorious potentials of porphyrinoids. In 2003, Furuta et al. have combined these two porphyrinoids by synthesizing expanded NCPs such as doubly N-confused [26]dioxohexaphyrins(1.1.1.1.1.1) 1 and doubly N-confused and ring-contracted [26]dioxohexaphyrins(1.1.1.1.1.0) 2 (Fig. 1 ) [10] , [11] , [12] , [13] , [14] . These molecules were synthesized by acid-catalyzed condensation reactions and the lactam units were formed via facile oxidation of the N-confused pyrroles. The oxidized N-confused pyrrole units in 1 and 2 have been shown to be quite effective for the coordination of transition metal ions, allowing for the synthesis of various metal complexes. On the other hand, attempts to synthesize doubly N-confused non-oxo [26]hexaphyrin metal complexes ended in very low yields [15] . In addition, these synthetic methods provided only thermodynamically stable aromatic products. As a rare example, Furuta et al. reported that electrochemical oxidation of 2Cu led to the generation of 24π-antiaromatic species [14] , but antiaromatic expanded NCP has been never isolated before. In this work, we report the serendipitous synthesis of d oubly N - c onfused and r ing- c ontracted (DNCRC) [24]hexaphyrin(1.1.0.1.1.0) Pd II complexes 8 and 9 by Pd-catalyzed self-coupling reaction of α , α -dibromotripyrrin 3b . Fig. 1: Structures of N-confused hexaphyrins. Structures of doubly N-confused [26]dioxohexaphyrins(1.1.1.1.1.1) 1 , doubly N-confused and singly ring-contracted [26]dioxohexaphyrins(1.1.1.1.1.0) 2 , and its Cu II complex 2Cu . Full size image With the aim to synthesize m -benziporphyrin(1.1.0.0) 5 , we attempted the cyclization reaction of α , α ’-diboryltripyrrane 3a with 1,3-dibromo-4-methoxybenzene under the usual Suzuki–Miyaura coupling conditions (Pd 2 (dba) 3 , X-phos, Cs 2 CO 3 , CsF, and toluene/DMF). In addition to the target 5 [16] which was actually obtained in 5% yield, we isolated dark green product 6 in ca. 1% (Fig. 2 ). Fortunately, the structure of 6 has been revealed by X-ray analysis to be a symmetric and planar [18]triphyrin(5.1.1) with a small mean-plane deviation (MPD) of 0.26 Å (Fig. 3a, b ). The carbonyl oxygen atom is hydrogen bonded with the two adjacent pyrrolic NH groups and the C=O bond length is 1.288(7) Å, being distinctly longer than those of usual ketones (1.23 Å) [17] , [18] . This structural feature suggests a significant contribution of a dipolar resonance state. The 1 H NMR spectrum of 6 shows a singlet at 9.74 ppm due to the vinylic proton, two doublets at 8.36 and 8.08 ppm ( J = 4.0 Hz) and a singlet at 8.31 ppm due to the pyrrolic protons, and signals due to the NH protons at 3.89 (2H) and −4.13 (1H) ppm, suggesting a distinct diatropic ring current, reflecting its 18 π -electronic circuit. The absorption spectrum of 6 shows a split Soret-like band at 419 and 444 nm and vibronic-structured Q-like bands as characteristic features of aromatic porphyrinoids (Fig. 4 ). Further, 6 displays vibronic-structured fluorescence at 652 and 721 nm with a high quantum yield of Φ F = 0.48. These data strongly indicate that 6 is an aromatic tripyrrolic porphyrinoid. Actually, the calculated NICS values are negative (−12.15 ppm) inside the macrocycle. Fig. 2: Synthesis of compounds 5 and 6. Dba = dibenzylideneacetone, Mes = 2,4,6-trimethylphenyl, Bpin = pinacolatoboryl, DDQ = 2,3-dicyano-5,6-dichlorobenzoquinone. Full size image Fig. 3: X-ray crystal structures of 6 and 7. a Top view of 6 , b side view of 6 , c top view of 7 , d side view of 7 . Ellipsoids are drawn at the 30% probability level. All hydrogen atoms except those connected to N and O atoms are omitted for clarity. Carbon atom, black ellipsoid; nitrogen atom, blue; palladium atom, orange; oxygen atom, red; hydrogen atom small black ball (These instructions are omitted in the following figures for clarity). Full size image Fig. 4: UV–Vis absorption spectrum and fluorescence spectrum of 6 in CH 2 Cl 2 . Solid line, absorption spectrum; dash line, fluorescence spectrum. Full size image Since 6 can be regarded as a cyclized product of 3a and dibenzalacetone, we examined the reaction of only 3a under the same conditions, which actually gave 6 in 5–8% yield. In the next step, we examined the reaction of 3a with dibenzalacetone and found that 6 was obtained in 8.8% under conditions (3 eq. dibenzalacetone, 0.4 equiv PPh 3 , 2 mol% Pd 2 (dba) 3 , 2 eq. Cs 2 CO 3 , CsF). In continuation of this study, we examined the reaction of 1,14-dibromotripyrrin 3b under the similar Suzuki–Miyaura coupling conditions (X-phos, Cs 2 CO 3 , CsF, Pd 2 (dba) 3 , toluene, DMF, reflux, 48 h), and found quite unexpectedly that [24]hexaphyrin Pd-complexes 8 (9%) and 9 (10%) were obtained along with 6 (1%) and tripyrrolic compound 7 (2%) (Fig. 5 ). The structure of 7 has been revealed by X-ray analysis (Fig. 3c, d ) to be a coupling product of 3 and dibenzalacetone. Fig. 5: Synthesis of compounds 6, 7, 8, 9, 9Pd, 9Ni and 9Cu. Reaction conditions: a X-phos, Cs 2 CO 3 , CsF, Pd 2 (dba) 3 , toluene, DMF, reflux, 48 h; b M(OAc) 2 , NaOAc, CHCl 3 , MeOH, reflux. Full size image The parent ion peaks of 8 and 9 were observed at m/z = 1120.2568 (calcd for (C 64 H 54 N 6 Pd 2 ) + = 1120.2504 ([ M ] + )) and at m/z = 1030.3687 (calcd for (C 64 H 56 N 2 Pd) + = 1030.3566 ([ M ] + )) by high-resolution MALDI-TOF mass measurement. Both the structures of 8 and 9 have been revealed to be d oubly N - c onfused and r ing- c ontracted (DNCRC) [24]hexaphyrins(1.1.0.1.1.0) by X-ray analysis (Fig. 6 ). Product 8 is a nonoxo DNCRC [24]hexaphyrin, displaying a very planar structure with a small MPD (0.04 Å), in which the two Pd metals are coordinated with the three pyrrolic nitrogen atoms and one α -carbon of the N-confused pyrrole with a bond distance of 2.002(4) Å for Pd1–N1, 2.027(5) Å for Pd1–N2, 1.959(5) Å for Pd1–N3, and 1.972(5) Å for Pd1–C. As compared with the previously reported Pd II complexes of NCPs that showed bond distances of Pd–C (2.002–2.003 Å) and Pd–N (2.003 Å) [19] , [20] , [21] , Pd1–N2 and Pd1–C bond lengths are distinctly shorter. The 1 H NMR spectrum of 8 shows signals due to the β -pyrrolic protons as a singlet at 4.01 ppm and two doublets at 4.85 and 5.10 ppm ( J = 4.5 Hz) and at 5.25 and 5.30 ppm ( J = 4.5 Hz), indicating a weak but distinct paratropic ring current. The absorption spectrum of 8 is ill-defined, showing peaks at 396, 502, 618, 687, 763, 1015, and 1176 nm. The HOMA value was calculated to be 0.51 based on the crystallographic data, and the NICS value at the center of the molecule was calculated to be 5.41, indicating the weak antiaromatic character of 8 . In addition, the ACID plot (see Supplementary Fig. 58 ) of complex 8 displayed a continuous paratropic ring current, being consistent with the NICS(0) value. Fig. 6: X-ray crystal structures of 8, 9 and 9Pd. a Top view of 8 , b side view of 8 , c top view of 9 , d side view of 9 , e top view of 9Pd , f side view of 9Pd . Ellipsoids are drawn at the 30% probability level. All hydrogen atoms except those connected to N atoms are omitted for clarity. Full size image The structure of 9 has been determined by X-ray diffraction analysis to be a DNCRC keto tautomer, in which one α -position of the N-confused pyrrole is oxidized. Unfortunately, the serious disorder impeded a detailed analysis of the structure. The 1 H NMR spectrum of 9 displays two signals due to the inner NH protons at 21.89 and 19.85 ppm and those in the range of 5.22–3.79 ppm due to the pyrrolic β - protons, clearly indicating its paratropic ring current and thus antiaromatic character. Judging from these chemical shifts, it is conceivable that the antiaromatic character of 9 is slightly larger as compared with 8 . The NICS value of 9 was calculated to be 10.43, which is larger than that of 8 . Importantly, 8 and 9 are stable antiaromatic N-confused expanded porphyrins. Hexaphyrin 9 has been demonstrated to be a nice platform to form bis-metalated complexes. Actually, complexes 9Pd , 9Ni , and 9Cu were readily obtained in 80%, 95%, and 85% upon complexation with Pd II , Ni II , and Cu II ions, respectively. The 1 H NMR spectra of 9Pd and 9Ni show signals due to the peripheral β -protons in the range of 5.40–4.09 and 5.20–3.77 ppm, respectively, revealing paratropic rings current comparable to that in 9 . The structure of 9Pd has been revealed by X-ray analysis, displaying a slightly curved structure with a large MPD (0.36 Å). Pd1 is coordinated with the three pyrrolic nitrogen atoms and one α -carbon of the N-confused pyrrole with a bond length of 2.034(6) Å for Pd1–N1, 2.029(5) Å for Pd1–N2, 1.956(5) Å for Pd1–N3, and 2.073(6) Å for Pd1–C. Pd2 is coordinated with the three pyrrolic nitrogen atoms and one oxygen atom with a bond length of 1.967(5) Å for Pd2–N4, 1.962(5) Å for Pd2–N5, 1.968(5) Å for Pd2–N6, and 2.002(5) Å for Pd2–O1. The absorption spectra of 8 , 9 , 9Pd , 9Ni , and 9Cu are shown in Fig. 7a . Characteristically, all these DNCRC [24]hexaphyrin complexes show ill-defined Soret bands and weak bands in the range of 800–1400 nm in line with their antiaromatic properties. Judging from the most red-shifted bands, the optical HOMO–LUMO gaps have been estimated to be 1.05, 1.15, 1.12, 1.05, and 1.08 eV for 8 , 9 , 9Pd , 9Ni , and 9Cu , respectively. Fig. 7: Absorption spectra of 8, 9, 9Cu, 9Pd, 9Ni, 10 and 12 in CH 2 Cl 2 . a UV–Vis absorption spectra of 8 , 9 , 9Pd , 9Ni and 9Cu in CH 2 Cl 2 ; b UV–Vis absorption spectra of 8 , 10 and 12 in CH 2 Cl 2 . 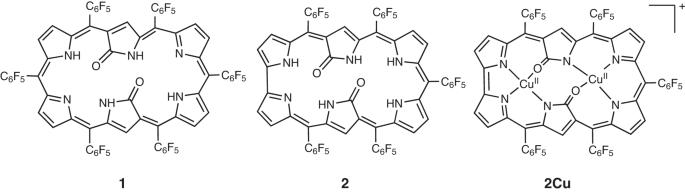Fig. 1: Structures of N-confused hexaphyrins. Structures of doubly N-confused [26]dioxohexaphyrins(1.1.1.1.1.1)1, doubly N-confused and singly ring-contracted [26]dioxohexaphyrins(1.1.1.1.1.0)2, and its CuIIcomplex2Cu. Full size image Cyclic voltammetry (CV) and differential-pulse voltammetry (DPV) experiments were conducted and the redox potentials are summarized in Table 1 . Table 1 Electrochemical properties of 8 , 9 , 9 Pd , 9Ni , and 9Cu in CH 2 Cl 2 with 0.1 M n -Bu 4 NPF 6 a Full size table The electrochemical properties were investigated by cyclic voltammetry and differential pulse voltammetry. Complex 8 showed reversible oxidation waves at 0.65 and 0.18 V and reduction waves at −1.05, −1.52, and −1.79 V, indicating the HOMO–LUMO gap to be 1.23 eV. Complexes 9 , 9 Pd , 9Ni , and 9Cu showed HOMO–LUMO gaps of 1.12, 1.19, 1.20, and 1.15 eV, respectively, roughly matching with the optical HOMO-LUMO gaps. Further fabrications of 8 were attempted. Monobromide 8a was obtained in 78% yield by treating 8 with 1 equiv. NBS at 0 °C (Fig. 8 ). The parent ion peak of 8a was observed at m/z = 1196.1615 (calcd for (C 64 H 53 BrN 6 Pd 2 ) + = 1196.1601 ([ M ] + )) and its 1 H NMR spectrum showed nine peaks at 5.23–4.05 ppm, indicating an asymmetric substitution. Subsequently, directly β -to- β linked DNCRC [24]hexaphyrin dimer 10 was successfully obtained by reductive coupling of 8a with Ni(cod) 2 in 61% yield. The parent ion peak of 10 was observed at m/z = 2234.4843 (calcd for (C 128 H 106 N 12 Pd 4 ) + = 2234.4862 ([ M ] + )). The 1 H NMR spectrum of 10 exhibited three singlets at 4.30, 3.91, and 3.74 ppm and three pairs of doublets in the range of 5.13–4.69 ppm. The structure of 10 has been confirmed by X-ray analysis as shown in Fig. 9 . The dihedral angle between the two hexaphyrins is 54.2° and the bond length of the connecting C–C is 1.48 (1) Å. The first oxidation potentials of 10 were split at 0.31 and 0.15 V, indicating the electronic interaction between the two DNCRC [24]hexaphyrin units. Fig. 8: Synthesis of compounds 8a, 8b, 10 and 12. Reaction conditions: a NBS (1.0 equiv or 2.0 equiv. ), 0 °C, CHCl 3 ; b Ni(cod)2 (1.0 equiv), 2,2’-bipyridine (1.0 equiv), reflux, 24 h; c SPhos Pd G2 (10 mol %), K 3 PO 4 (5.0 equiv. ), THF/H 2 O = 20:1, reflux, 36 h. Full size image Fig. 9: X-ray crystal structures of 10 and 12. a Top view of 10 , b side view of 10 , c top view of 12 , and d side view of 12 . Ellipsoids are drawn at the 30% probability level. All hydrogen atoms are omitted for clarity. Meso -substituents of porphyrin parts are omitted for clarity. Nickel atom, green. Full size image Dibromide 8b was obtained in 86% yield by treating 8 with 2 equiv. NBS at 0 °C. The parent ion peak of 8b was observed at m/z = 1274.0660 (calcd for (C 64 H 52 Br 2 N 6 Pd 2 ) + = 1274.0701 ([ M ] + )) and its 1 H NMR spectrum showed two doublets at 5.22 and 4.84 ppm ( J = 4.7 Hz) and two singlets at 5.20 and 4.23 ppm, indicating a symmetric substitution. The single-crystal structure of 8b was also determined by X-ray diffraction analysis, which shows its centrosymmetric dibromide feature. Finally, the Suzuki–Miyaura coupling reaction between 8b and 5-boryl-10,15,20-triarylporphyrinato Ni II 11 gave Ni II porphyrin-DNCRC [24hexaphyrin-Ni II porphyrin triad 12 , in 43% yield. The parent ion peak of 12 was observed at m/z = 2975.2621 (calcd for (C 188 H 194 N 14 Ni 2 Pd 2 ) + = 2975.2429 ([ M ] + )). The 1 H NMR spectrum showed two singlets at 5.94 and 5.58 ppm and a pair of doublets at 5.19 and 4.70 ppm, revealing its symmetric structure. The dihedral angle between the hexaphyrin and Ni II porphyrin is 58.9° and the newly formed C–C bonds are 1.47 (1) Å long. The absorption spectra of 8 , 10 , and 12 are shown in Fig. 7b . Dimer 10 shows bands at 395, 503, 635, 712, and 796 nm along with a weak tail. The three bands observed at longer wavelengths are considerably red-shifted in comparison to those of 8 . Triad 12 displays a Soret band of the Ni II porphyrins at 416 nm. A red-shifted band of the DNCRC [24]hexaphyrin observed at 792 nm suggests its substantial electronic interaction with the Ni II porphyrin. In summary, 1,14-dibromotripyrrin 3b underwent a self-coupling reaction under Pd-catalyzed Suzuki–Miyaura coupling conditions, giving DNCRC [24]hexaphyrin(1.1.0.1.1.0) Pd II complexes 8 and 9 , along with 1,14-dibromotripyrrin–benzalacetone coupled products 6 and 7 . While triphyrin 6 is an aromatic [18] triphyrin(5.1.1), DNCRC [24]hexaphyrins 8 and 9 are stable antiaromatic expanded NCP showing paratropic ring currents, ill-defined absorption spectra with red-shifted weak absorption bands, and small HOMO–LUMO gaps. Monobromide 8a was reductively dimerized to give 10 and dibromide 8b was coupled with 11 to give Ni II porphyrin-DNCRC [24hexaphyrin-Ni II porphyrin triad 12 . Materials and characterization 1 H NMR spectra (500 MHz) were taken on a Bruker ADVANCE-500 spectrometer, and chemical shifts were reported as the delta scale in ppm relative to CHCl 3 ( δ = 7.260 ppm) as an internal reference. UV/Vis absorption spectra were recorded on a Shimadzu UV-3600 spectrometer. MALDI-TOF mass spectra were obtained with a Bruker ultrafleXtreme MALDI-TOF/TOF spectrometer with trans -2-[3-(4- tert -Butylphenyl)-2-methyl-2-propenylidene]malononitrile (DCTB) as a matrix. X-ray data were taken on an Agilent Supernova X-ray diffractometer equipped with a large area CCD detector. Redox potentials were measured by cyclic voltammetry on a CHI900 scanning electrochemical microscope. Toluene and THF were distilled after refluxing with Na and benzophenone ketyl indicator under an argon atmosphere and stored over 3 Å molecular sieves in a glovebox for at least 12 h prior to use. DMF was refluxed with CaH 2 under an argon atmosphere for at least 3 h and distilled prior to use. Unless otherwise noted, materials obtained from commercial suppliers were used without further purification. Synthesis of 5 and 6 A suspension of 1,14-diboryltripyrrane 3a (214.0 mg, 0.30 mmol), 2,4-dibromo-1-methoxybenzene (53.2 mg, 0.20 mmol), Pd 2 (dba) 3 (18.3 mg, 0.02 mmol), X-Phos (38.1 mg, 0.08 mmol), Cs 2 CO 3 (130.3 mg, 0.40 mmol), and CsF (60.7 mg, 0.40 mmol) in toluene/DMF suspension (4 mL/2 mL) was degassed through three freeze–pump–thaw cycles, and the reaction flask was purged with argon. The resulting mixture was refluxed for 48 h. The reaction mixture was diluted with CHCl 3 . The organic layer was separated and washed with water, and dried over anhydrous sodium sulfate. Evaporation of the solvent followed by silica-gel column chromatography (eluent: CH 2 Cl 2 / n -hexane = 1:4, v/v) and recrystallization with CH 2 Cl 2 /MeOH gave 5 as green solids (5.6 mg, 0.010 mmol, 5% yield) and 6 as dark green solids (1.4 mg, 0.0020 mmol, 1% yield). 5 : 1 H NMR (500 MHz, CDCl 3 ) δ = 17.85 (br, 1H, N-H), 12.50 (d, 1H, J = 2.0 Hz, Ph-H), 7.36 (dd, 1H, Ph-H), 6.87 (s, 4H, Mes- m -H), 6.69 (d, 1H, J = 4.5 Hz, β -H), 6.66 (d, 1H, J = 4.5 Hz, Ph-H), 6.58 (d, 1H, J = 4.5 Hz, β -H), 6.48 (d, 1H, J = 4.5 Hz, β -H), 6.46 (d, 1H, J = 4.5 Hz, β -H), 5.57 (m, 2H, β -H), 2.87 (s, 3H, OMe-H), 2.30 (s, 6H, Me-H) and 2.16 (s, 12H, Me-H) ppm. HR-MS (MALDI-TOF-MS): m/z = 561.2794, calcd for (C 39 H 35 N 3 O) + = 561.2775 ([ M ] + ). 6 : 1 H NMR (500 MHz, CDCl 3 ) δ = 9.74 (s, 2H, vinyl-H), 8.36 (d, J = 4.0 Hz, 2H, β -H), 8.31 (s, 2H, β -H), 8.20 (d, J = 7.2 Hz, 4H, Ph-H), 8.08 (dd, J = 4.0, 1.5 Hz, 2H, β -H), 7.73 (t, 4H, Ph-H), 7.67 (t, J = 6.0 Hz, 2H, Ph-H), 7.28 (s, 4H, Mes- m -H), 3.87 (s, 2H, N-H), 2.63 (br, 6H, Me-H), 1.89 (br, 12H, Me-H) and −4.13(s, 1H, N-H) ppm. 13 C NMR (126 MHz, CDCl 3 ) δ = 166.7, 145.4, 139.8, 137.8, 137.6, 137.1, 134.8, 134.6, 132.7, 132.6, 128.2, 128.0, 127.9, 127.5, 127.1, 123.8, 123.4, 122.0, 106.8, 21.6 and 21.1 ppm. UV/Vis (CH 2 Cl 2 ): λ max ( ε [M −1 cm −1 ]) = 419 (21,000), 444 (25,000), and 652(6300) nm. HR-MS (MALDI-TOF-MS): m/z = 689.3441, calcd for (C 49 H 43 N 3 O) + = 689.3401 ([ M ] + ). Synthesis of 6, 7, 8 and 9 A suspension of 1,14-dibromotripyrrin (100.0 mg, 0.16 mmol), Pd 2 (dba) 3 (50.0 mg, 0.05 mmol), X-Phos (38.1 mg, 0.08 mmol), Cs 2 CO 3 (130.3 mg, 0.40 mmol), and CsF (60.7 mg, 0.40 mmol) in toluene/DMF (4 mL/2 mL) was degassed through three freeze–pump–thaw cycles, and the reaction flask was purged with argon. The resulting mixture was stirred at reflux for 48 h. The reaction mixture was diluted with CHCl 3 . The organic layer was separated and washed with water, and dried over anhydrous sodium sulfate. Evaporation of the solvent followed by silica-gel column chromatography (eluent: CH 2 Cl 2 / n -hexane = 1:3, v/v) and recrystallization with CH 2 Cl 2 /MeOH gave 6 as dark green solids (1.10 mg, 0.0016 mmol, 1% yield), 7 as blue solids (2.4 mg, 0.003 mmol, 2% yield), 8 as gray-green solids (8.4 mg, 0.0075 mmol, 9% yield), and 9 as emerald green solids (5.2 mg, 0.005 mmol, 10% yield). 7 : 1 H NMR (500 MHz, CDCl 3 ) δ = 17.17 (br, 1H, OH), 7.29 (d, J = 7.5 Hz, 2H, Ph- o -H), 7.13-7.08 (m, 5H, Ph-H), 7.04 (t, J = 7.1 Hz, 1H, Ph- p -H), 6.99 (d, 2H, J = 7.5 Hz, Ph- o -H), 6.91 (s, 1H, Mes- m -H), 6.89 (s, 1H, Mes- m -H), 6.88 (s, 1H, Mes- m -H), 6.87 (s, 1H, Mes- m -H), 6.60–6.59 (m, 2H, β -H), 6.51 (d, J = 4.5 Hz, 1H, β -H), 6.26 (d, J = 4.3 Hz, 1H, β -H), 6.24 (d, J = 5.0 Hz, 1H, β -H), 5.91 (d, J = 4.3 Hz, 1H, β -H), 5.68 (d, J = 3.0 Hz, 1H, sp 3 C-H), 4.23 (d, J = 7.7 Hz, 1H, sp 3 C-H), 3.25 (dd, J = 16.5, 7.8 Hz, 1H, sp 3 C-H), 2.63 (dd, J = 16.5, 3.1 Hz, 1H, sp 3 C-H), 2.34 (s, 3H, Me-H), 2.32 (s, 3H, Me-H), 2.18 (s, 3H, Me-H), 2.09 (s, 3H, Me-H), 2.05 (s, 3H, Me-H) and 1.96 (s, 3H, Me-H) ppm. 13 C NMR (126 MHz, CDCl 3 ) δ = 179.7, 179.0, 146.9, 144.6, 141.2, 141.0, 139.7, 139.5, 137.7, 137.6, 137.54, 137.47, 137.0, 136.9, 134.2, 133.8, 133.6, 131.7, 130.0, 128.51, 128.46, 128.2, 128.1, 128.0, 127.8, 126.8, 126.4, 122.2, 121.9, 118.7, 64.4, 54.6, 54.2, 45.9, 21.3, 21.2, 20.7, 20.4(2C) and 20.2 ppm. (The absence of some peaks in 13 C NMR may be due to overlapping.) UV/Vis (CH 2 Cl 2 ): λ max ( ε [M −1 cm −1 ]) = 355 (21,100), 400 (26,500), and 667 (6600) nm. HR-MS (MALDI-TOF-MS): m/z = 811.2408, calcd for (C 49 H 43 N 3 O 2 Pd) + = 811.2402 ([ M ] + ). 8 : 1 H NMR (500 MHz, CDCl 3 ) δ = 6.72 (s, 4H, Mes- m -H), 6.68 (s, 4H, Mes- m -H), 5.20 (d, J = 4.5 Hz, 2H, β -H), 5.18 (d, J = 4.5 Hz, 2H, β -H), 5.12 (d, J = 4.5 Hz, 2H, β -H), 4.80 (d, J = 4.5 Hz, 2H, β -H), 4.02 (s, 2H, β -H), 2.25 (s, 12H, Me-H), and 2.18–2.16 (m, 24H, Me-H). 13 C NMR (126 MHz, CDCl 3 ) δ = 223.8, 161.5, 153.1, 152.0, 149.5, 148.3, 143.9, 138.5, 137.3, 137.1, 136.1, 132.5, 131.9, 131.8, 131.6, 128.5, 127.9, 127.8, 121.2, 120.4, 114.3, 29.8, 21.0, 19.9, and 19.4 ppm. (The absence of some peaks in 13 C NMR may be due to overlapping). UV/Vis (CH 2 Cl 2 ): λ max ( ε [M −1 cm −1 ]) = 340 (25,200), 396 (44,100), 502 (28,800), 618 (35,300), 690 (7100), 763 (7600), and 1082 (100) nm. HR-MS (MALDI-TOF-MS): m/z = 1120.2568, calcd for (C 64 H 54 N 6 Pd 2 ) + = 1120.2504 ([ M ] + ). 9 : 1 H NMR (500 MHz, CDCl 3 ) δ = 21.89 (s, 1H, N-H), 19.85 (s, 1H, N-H), 6.68-6.64 (m, 8H, Mes- m -H), 5.22 (d, J = 4.5 Hz, 1H, β -H), 5.13 (d, J = 4.5 Hz, 1H, β -H), 5.10 (dd, J = 4.5, 2.0 Hz, 1H, β -H), 5.07 (dd, J = 4.5, 2.0 Hz, 1H, β -H), 5.02 (d, J = 4.5 Hz, 1H, β -H), 4.88 (d, J = 4.5 Hz, 1H, β -H), 4.73 (d, J = 4.5 Hz, 1H, β -H), 4.62 (d, J = 4.5 Hz, 1H, β -H), 4.30 (s, 1H, β -H), 3.79 (s,1H, β -H) and 2.22-2.12 (m, 36H, Me-H). 13 C NMR (126 MHz, CDCl 3 ) δ = 215.8, 187.1, 166.2, 157.6, 155.8, 155.4, 151.3, 149.7, 140.3, 137.64, 137.56, 137.1, 137.0, 135.9, 135.7, 132.8, 132.1, 131.9, 131.4, 130.7, 128.4, 128.0, 127.9, 126.7, 125.7, 124.4, 123.8, 123.0, 120.3, 116.0, 113.2, 110.7, 100.0, 29.7, 21.0, 20.0, 19.5, and 19.1 ppm. (The absence of some peaks in 13 C NMR may be due to overlapping.) UV/Vis (CH 2 Cl 2 ): λ max ( ε [M −1 cm −1 ]) = 364 (29,400), 487 (26,700), 628 (21,200), 987 (200), and 1119 (200) nm. HR-MS (MALDI-TOF-MS): m/z = 1030.3687, calcd for (C 64 H 56 N 6 OPd) + = 1030.3566 ([ M ] + ). Synthesis of 8a A solution of NBS (3.2 mg, 0.018 mmol) in CHCl 3 (10 mL) was added to a solution of 8 (20.0 mg, 0.018 mmol) in CHCl 3 (10 mL) dropwise at 0 °C. After the consumption of 8 was confirmed by TLC monitoring, the reaction mixture was diluted with CHCl 3 . The organic layer was separated and washed with water, and dried over anhydrous sodium sulfate, evaporation of the solvent was followed by silica-gel column chromatography (eluent: CH 2 Cl 2 / n -hexane = 1:4, v/v) and recrystallization with CH 2 Cl 2 /MeOH. 8a was obtained as grass-green solids (16.7 mg, 0.014 mmol, 78% yield). 8a : 1 H NMR (500 MHz, CDCl 3 ) δ = 6.71 (s, 4H, Mes- m -H), 6.67 (s, 4H, Mes- m -H), 5.23 (d, J = 4.5 Hz, 1H, β -H), 5.21 (d, J = 4.5 Hz, 1H, β -H), 5.15 (s, 1H, β -H), 5.14 (s, 1H, β -H), 5.13 (s, 1H, β -H), 4.81-4.80 (m, 2H, β -H), 4.17 (s, 1H, β -H), 4.05 (s, 1H, β -H), 2.22 (br, 6H, Me-H), 2.21 (br, 6H, Me-H), and 2.18-2.15 (m 24H, Me-H). HR-MS (MALDI-TOF-MS): m/z = 1196.1615, calcd for (C 64 H 53 BrN 6 Pd 2 ) + = 1196.1601 ([ M ] + ). Synthesis of 8b A solution of NBS (6.4 mg, 0.036 mmol) CHCl 3 (10 mL) was added to a solution of 8 (20.0 mg, 0.018 mmol) in CHCl 3 (20 mL) dropwise at 0 °C. After the consumption of 8 and 8a was confirmed by TLC monitoring, the reaction mixture was diluted with CHCl 3 . The organic layer was separated and washed with water, and dried over anhydrous sodium sulfate, Evaporation of the solvent was followed by silica-gel column chromatography (eluent: CH 2 Cl 2 / n -hexane = 1:4, v/v) and recrystallization with CH 2 Cl 2 /MeOH gave 8b as grass green solids (19.7 mg, 0.016 mmol, 86% yield). 8b : 1 H NMR (500 MHz, CDCl 3 ) δ = 6.72 (s, 4H, Mes- m -H), 6.68 (s, 4H, Mes- m -H), 5.21 (d, J = 4.5 Hz, 2H, β -H), 5.20 (s, 2H, β -H), 4.84 (d, J = 4.5 Hz, 2H, β -H), 4.22 (s, 2H, β -H), 2.22 (br, 12H, Me-H), 2.18 (br, 6H, Me-H), and 2.16 (br, 18H, Me-H). HR-MS (MALDI-TOF-MS): m/z = 1274.0660, calcd for (C 64 H 52 Br 2 N 6 Pd 2 ) + = 1274.0701 ([ M ] + ). Synthesis of 9Cu A suspension of 9 (20.0 mg, 0.019 mmol), Cu(OAc) 2 (37.8 mg, 0.19 mmol), and NaOAc (15.6 mg, 0.19 mmol) in CHCl 3 /MeOH (20 mL/10 mL) was stirred at 65 °C overnight. The solvent was removed under reduced pressure. The product was separated by silica-gel column chromatography (eluent:CH 2 Cl 2 / n -hexane = 1:1, v/v) and recrystallization with CH 2 Cl 2 /MeOH gave 9Cu as brown crystals (17.6 mg, 0.016 mmol, 85% yield). UV/Vis (CH 2 Cl 2 ): λ max ( ε [M −1 cm −1 ]) = 368 (38,200), 472 (33,300), 630 (24,000), 994 (300) and 1166 (200) nm. HR-MS (MALDI-TOF-MS): m/z = 1091.2730, calcd for (C 64 H 54 CuN 6 OPd) + = 1091.2702([ M + H] + ). Synthesis of 9Pd and 9Ni By following the method used for the synthesis of 9Cu — 9Pd and 9Ni were synthesized upon treatment with Pd(OAc) 2 and Ni(OAc) 2 ·4H 2 O in 80% and 95% yields. 9Pd : 1 H NMR (500 MHz, CDCl 3 ) δ = 6.90 (br, 1H, Mes- m -H), 6.76 (br, 1H, Mes- m -H), 6.73 (br, 1H, Mes- m -H), 6.72 (br, 2H, Mes- m -H), 6.69 (br, 1H, Mes- m -H), 6.65 (br, 2H, Mes- m -H), 5.40 (d, J = 4.6 Hz, 1H, β -H), 5.38–5.33 (m, 4H, β -H), 5.10 (d, J = 4.6 Hz, 1H, β -H), 5.00 (d, J = 4.6 Hz, 1H, β -H), 4.86–4.83 (m, 2H, β -H), 4.09 (s, 1H, β -H), 2.85 (s, 3H, Me-H), 2.37 (s, 3H, Me-H), 2.31 (s, 3H, Me-H), 2.22 (s, 3H, Me-H), 2.20 (s, 3H, Me-H), 2.19 (s, 9H, Me-H), 2.16 (s, 3H, Me-H), 2.02 (s, 3H, Me-H), 1.99 (s, 3H, Me-H), and 1.65 (s, 3H, Me-H). 13 C NMR (126 MHz, CDCl 3 ) δ = 212.4, 184.4, 159.0, 158.0, 154.0, 150.4, 150.2, 150.0, 147.7, 145.9, 142.8, 141.7, 137.7, 137.4, 137.3, 137.2, 136.8, 136.5, 136.3, 136.3, 136.1, 136.1, 136.0, 136.0, 132.2, 131.6, 131.2, 131.2, 129.9, 129.9, 129.3, 128.2, 128.0, 127.8, 127.8, 127.7, 124.5, 121.5, 120.3, 118.0, 116.8, 113.2, 21.0, 21.0, 20.8, 20.2, 19.7, 19.6 and 19.4 ppm. (The absence of some peaks in 13 C NMR may be due to overlapping.) UV/Vis (CH 2 Cl 2 ): λ max ( ε [M −1 cm −1 ]) = 411 (26,600), 316 (5700) and 490 (38,000) nm. HR-MS (MALDI-TOF-MS): m/z = 1136.2426, calcd for (C 64 H 54 N 6 OPd 2 ) + = 1136.2453 ([ M + H] + ). 9Ni : 1 H NMR (500 MHz, CDCl 3 ) δ = 6.89 (br, 1H, Mes- m -H), 6.70 (br, 1H, Mes- m -H), 6.68 (br, 1H, Mes- m -H), 6.68 (br, 1H, Mes- m -H), 6.65 (br, 1H, Mes- m -H), 6.63 (br, 1H, Mes- m -H), 6.60 (br, 2H, Mes- m -H), 5.20 (d, 1H, J = 4.6 Hz, β -H), 5.14-5.12 (m, 2H, β -H), 5.10 (d, 1H, J = 4.6 Hz, β -H), 5.07 (d, 1H, J = 4.6 Hz, β -H), 4.90 (d, 1H, J = 4.6 Hz, β -H), 4.83 (d, 1H, J = 4.6 Hz, β -H), 4.61-4.60 (m, 2H, β -H), 3.77 (s, β -H), 2.95 (s, 3H, Me-H), 2.23 (s, 3H, Me-H), 2.22 (s, 3H, Me-H), 2.20 (s, 3H, Me-H), 2.20 (s, 3H, Me-H), 2.18 (s, 3H, Me-H), 2.16 (s, 3H, Me-H), 2.15 (s, 3H, Me-H), 2.12 (s, 3H, Me-H), 2.10 (s, 3H, Me-H), 2.08 (s, 3H, Me-H) and 1.62 (s, 3H, Me-H). 13 C NMR (126 MHz, CDCl3) δ = 217.9, 187.1, 160.2, 158.7, 154.42, 154.39, 152.30, 152.0, 151.3, 147.6, 146.6, 144.1, 143.39, 139.8, 137.5, 137.3, 137.2, 136.0, 135.9, 132.0, 131.6, 131.4, 131.0, 130.2, 128.5, 128.2, 128.0, 127.9, 127.6, 122.6, 121.1, 119.9, 118.5, 113.2, 29.7, 21.0, 20.9, 20.8, 20.0, 19.8, 19.5, 19.4, 19.3 and 19.2 ppm. (The absence of some peaks in 13 C NMR may be due to overlapping.) UV/Vis (CH 2 Cl 2 ): λ max ( ε [M −1 cm −1 ]) = 393 (19,000), 836 (4000) and 931 (4600) nm. HR-MS (MALDI-TOF-MS): m / z = 1086.2635, calcd for (C 64 H 54 NiN 6 OPd) + = 1086.2758 ([ M ] + ). Synthesis of 10 A THF solution (5 mL) of 8a (20.0 mg, 0.017 mmol), Ni(cod) 2 (4.6 mg, 0.017 mmol), and 2,2’-bipyridine (2.7 mg, 0.017 mmol) in a 50 mL Schlenk tube was purged with argon. The mixture was refluxed for 24 h. The reaction mixture was diluted with CHCl 3 . The organic layer was separated and washed with water, and dried over anhydrous sodium sulfate. Evaporation of the solvent followed by silica-gel column chromatography (eluent: CH 2 Cl 2 / n -hexane = 1:3, v/v) and recrystallization with CH 2 Cl 2 /MeOH gave 10 as green solids (11.6 mg, 0.005 mmol, 61% yield). 10 : 1 H NMR (500 MHz, CDCl 3 ) δ = 6.81 (s, 2H, Mes- m -H), 6.70-6.69 (m, 8H, Mes- m -H), 6.62 (s, 2H, Mes- m -H), 6.59 (s, 2H, Mes- m -H), 5.13 (d, 2H, J = 4.5 Hz, β -H), 5.12 (d, 2H, J = 4.5 Hz, β -H), 5.08 (d, 2H, J = 4.5 Hz, β -H), 4.95 (d, 2H, J = 4.0 Hz, β -H), 4.70 (d, 2H, J = 4.5 Hz, β -H), 4.69 (d, 2H, J = 4.0 Hz, β -H), 4.30 (s, 2H, β -H), 3.91 (s, 2H, β -H), 3.74 (s, 2H, β -H), 2.59 (s, 6H, Me-H), 2.37 (s, 6H, Me-H), 2.23 (br, 18H, Me-H), 2.19 (br, 9H, Me-H), 2.17 (br, 9H, Me-H), 2.13 (br, 9H, Me-H), 2.12 (br, 9H, Me-H), 2.05 (s, 6H, Me-H) and 2.02 (s, 6H, Me-H). UV/Vis (CH 2 Cl 2 ): λ max ( ε [M −1 cm −1 ]) = 395 (72600), 503 (48,400), 635 (55,200), 712 (18,700), and 796 (30,700) nm. HR-MS (MALDI-TOF-MS): m/z = 2234.4843, calcd for (C 128 H 106 N 12 Pd 4 ) + = 2234.4862 ([ M ] + ). Synthesis of 12 A THF–H 2 O suspension (2 mL/0.1 mL) of 8b (20.0 mg, 0.016 mmol), 11 (34.0 mg, 0.032 mmol), Sphos Pd G2 (1.2 mg, 0.0016 mmol) and K 3 PO 4 (6.5 mg, 0.027 mmol) in a 50 mL Schlenk tube was purged with argon. The mixture was refluxed for 36 h. The reaction mixture was diluted with CHCl 3 . The organic layer was separated and washed with water, and dried over anhydrous sodium sulfate. Evaporation of the solvent followed by silica-gel column chromatography (eluent: CH 2 Cl 2 / n -hexane = 1:3, v/v) and recrystallization with CH 2 Cl 2 /MeOH gave 12 as dark green solids (20.5 mg, 0.007 mmol, 43% yield). 1 H NMR (500 MHz, CDCl 3 ) δ = 8.89 (d, J = 4.9 Hz, 4H, Por- β -H), 8.75 (dt, J = 8.6, 4.9 Hz, 12H, Por- β -H), 7.76 (s, 4H, Por-Ar-H), 7.71 (s, 2H, Por-Ar-H), 6.74 (s, 4H, Mes- m -H), 5.94 (s, 2H, β -H), 5.58 (s, 2H, β -H), 5.19 (d, J = 4.5 Hz, 2H, β -H), 4.70 (d, J = 4.5 Hz, 2H, β -H), 2.45 (s, 12H, Me-H), 2.14 (s, 6H, Me-H), 1.70 (s, 18H, Me-H) and 1.60 (s, 108H, t -Bu-H). 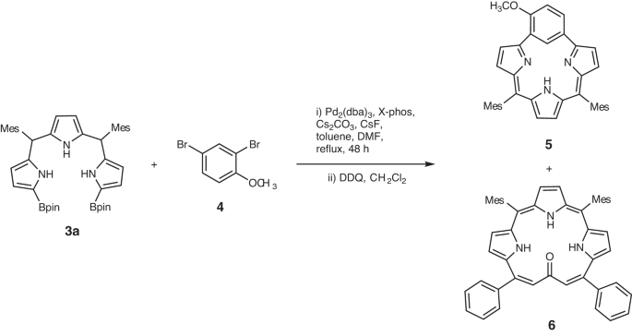Fig. 2: Synthesis of compounds 5 and 6. Dba = dibenzylideneacetone, Mes = 2,4,6-trimethylphenyl, Bpin = pinacolatoboryl, DDQ = 2,3-dicyano-5,6-dichlorobenzoquinone. 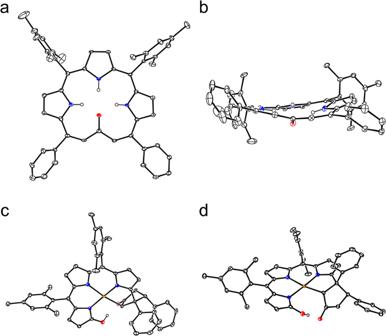Fig. 3: X-ray crystal structures of 6 and 7. aTop view of6,bside view of6,ctop view of7,dside view of7. Ellipsoids are drawn at the 30% probability level. All hydrogen atoms except those connected to N and O atoms are omitted for clarity. Carbon atom, black ellipsoid; nitrogen atom, blue; palladium atom, orange; oxygen atom, red; hydrogen atom small black ball (These instructions are omitted in the following figures for clarity). 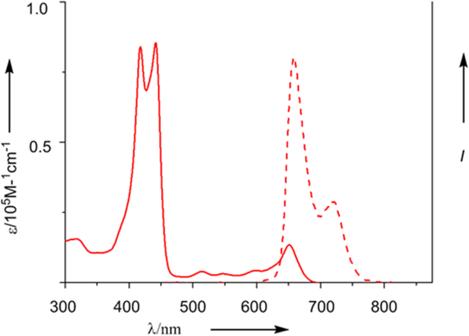Fig. 4: UV–Vis absorption spectrum and fluorescence spectrum of 6 in CH2Cl2. Solid line, absorption spectrum; dash line, fluorescence spectrum. UV/Vis (CH 2 Cl 2 ): λ max ( ε [M −1 cm −1 ]) = 416 (115,600), 636 (18,300), 714 (9300) and 792 (11,200) nm. 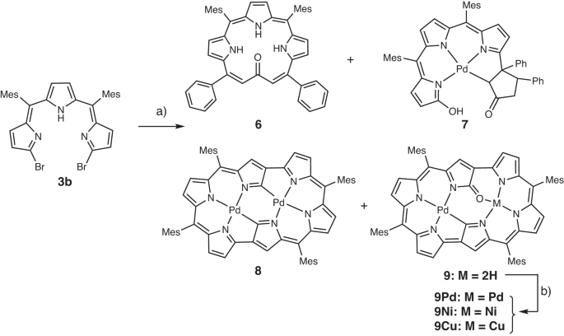Fig. 5: Synthesis of compounds 6, 7, 8, 9, 9Pd, 9Ni and 9Cu. Reaction conditions:aX-phos, Cs2CO3, CsF, Pd2(dba)3, toluene, DMF, reflux, 48 h;bM(OAc)2, NaOAc, CHCl3, MeOH, reflux. 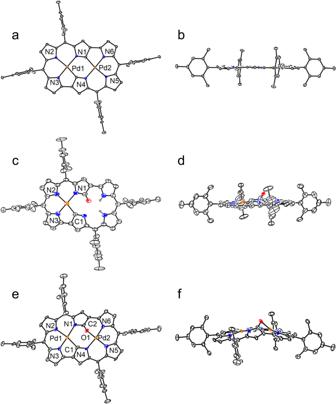Fig. 6: X-ray crystal structures of 8, 9 and 9Pd. aTop view of8,bside view of8,ctop view of9,dside view of9,etop view of9Pd,fside view of9Pd. Ellipsoids are drawn at the 30% probability level. All hydrogen atoms except those connected to N atoms are omitted for clarity. 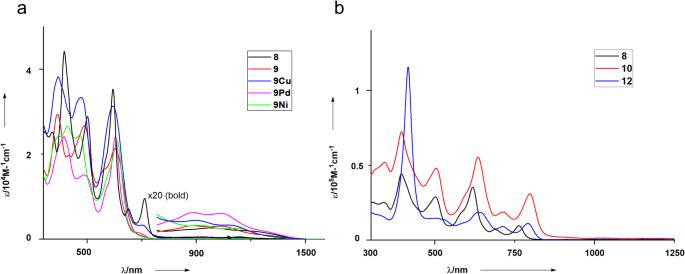Fig. 7: Absorption spectra of 8, 9, 9Cu, 9Pd, 9Ni, 10 and 12 in CH2Cl2. aUV–Vis absorption spectra of8,9,9Pd,9Niand9Cuin CH2Cl2;bUV–Vis absorption spectra of8,10and12in CH2Cl2. 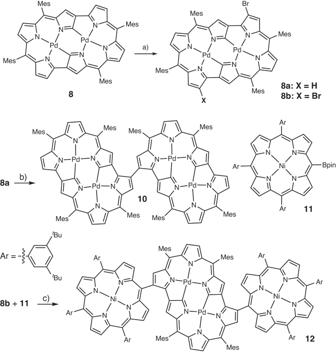Fig. 8: Synthesis of compounds 8a, 8b, 10 and 12. Reaction conditions:aNBS (1.0 equiv or 2.0 equiv.), 0 °C, CHCl3;bNi(cod)2 (1.0 equiv), 2,2’-bipyridine (1.0 equiv), reflux, 24 h;cSPhos Pd G2 (10 mol %), K3PO4(5.0 equiv.), THF/H2O = 20:1, reflux, 36 h. 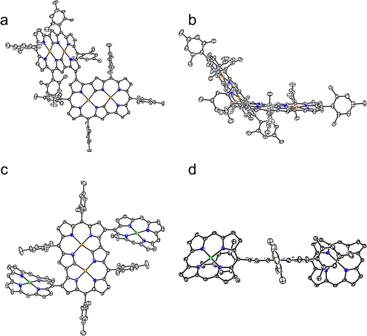Fig. 9: X-ray crystal structures of 10 and 12. aTop view of10,bside view of10,ctop view of12, anddside view of12. Ellipsoids are drawn at the 30% probability level. All hydrogen atoms are omitted for clarity.Meso-substituents of porphyrin parts are omitted for clarity. Nickel atom, green. HR-MS (MALDI-TOF-MS): m / z = 2975.2621, calcd for (C 188 H 194 N 14 Ni 2 Pd 2 ) + = 2975.2429 ([ M ] + ).